Hippos stem from the longest sequence of terrestrial cetartiodactyl evolution in Africa According to molecular data, hippopotamuses and cetaceans form a clade excluding other extant cetartiodactyls. Despite a wealth of spectacular specimens documenting cetacean evolution, this relationship remains poorly substantiated by the fossil record. Indeed, the evolutionary path leading from the hippo-cetacean ancestor to Hippopotamidae is plagued by missing fossil data and phylogenetic uncertainties. Only an origination within the extinct anthracotheres is compatible with molecular results, substantial filling of phyletic gaps and recent discoveries of early Miocene hippopotamids. Yet, the anthracothere stock that gave rise to Hippopotamidae has not been identified. Consequently, recent phylogenetic accounts do not properly integrate the anthracotheriid hypothesis, and relate Hippopotamidae to a stretched ghost lineage and/or close to Suina. Here we describe a new anthracothere from Lokone (Kenya) that unambiguously roots the Hippopotamidae into a well-identified group of bothriodontines, the first large mammals to invade Africa. The hippos are deeply anchored into the African Paleogene. Initially revealed by molecular data analyses, the exclusive clade grouping hippopotamuses with whales, dolphins and porpoises is also most often supported by combined analyses, as well as by some morphological analyses (see among others [1] , [2] , [3] ; and references herein). Regarding fossil support to this clade, early cetaceans are now known through an impressive fossil record documenting the acquisition of fully aquatic habits in this group [3] . However, few, much less spectacular fossil additions occurred for the hippopotamid branch, resulting in uncertainties on the nature and temporal placement of the hippopotamid-cetacean last common ancestor [2] . Apparently, these uncertainties sustained a diversity of opinions on the affinities of Hippopotamidae within fossil cetartiodactyls (for example, refs 2 , 3 , 4 , 5 , 6 , 7 , 8 ). Among these, some non-cladistic approaches are still radically in disagreement with molecular data [7] , [8] , whereas combined data set analyses have essentially maintained an unclear emergence of Hippopotamidae from an Oligocene ghost lineage, for example refs 3 , 4 , 9 . In fact, the integration of Miocene hippopotamid data into morphology-based cladistic analyses brought substantial support to a hippopotamid emergence among anthracotheres [10] , [11] . However, this approach did not succeed in precisely identifying the stem group of Hippopotamidae among anthracotheres. Boisserie et al. [2] (page 609) suggested that further resolution could come from further integration of the anthracothere fossil record, especially from the Oligocene of Africa. Unfortunately, Oligocene fossiliferous deposits are scarce on the Arabo-African continent. Discoveries of such deposits most often provide important evidence for the evolutionary history of mammals, in particular for primates [12] , [13] , [14] . And yet, despite several new early to late Oligocene sites found during the last decade [12] , [15] , [16] , [17] , [18] , [19] , the anthracothere diversity of Paleogene Arabo-Africa remained as described by Schmidt [20] and revised by Ducrocq [21] for the Fayum depression: four species of Bothriogenys and one of Qatraniodon [22] . An anthracothere, provisionally attributed to aff. Bothriogenys by Ducrocq et al. [19] , was discovered at Lokone, Turkana Basin and northern Kenya in deposits dated to the late early Oligocene or the early late Oligocene [19] . This anthracothere is the most abundant large mammal at Lokone, where it is associated with small taxa considered as relic species (for example, the phiomorph rodent Turkanamys hexalophus [23] and the parapithecid primate Lokonepithecus manai [13] ). We herein attribute this anthracothere to a new Oligocene genus and species that significantly improves our understanding of the anthracothere–hippopotamid relationships. It pushes back the evolutionary history of hippotamids in Africa to Paleogene adding the living hippotamuses to the long standing record of endemism of this continent. Systematic palaeontology of Epirigenys lokonensis Order Cetartiodactyla Montgelard, Catzeflys & Douzery 1997Suborder Cetancodonta, Arnason et al. , 2000Superfamily Hippopotamoidea, Gray, 1821 ( sensu Gentry & Hooker [24] ) Epirigenys nov. gen. Type species E. lokonensis nov gen nov sp Etymology The genus name is from ‘epiri’ the word for ‘hippopotamus’ in Turkana, and ‘genys’ a play on ancient Greek words for origin, source, lineage (-gen-) and for jaws (-genys). The species name refers to the discovery site of Lokone. Holotype KNM-LH 30375 (Lokone Hills, localities (Loc.) 1/2) left hemi mandible with P/3-M/2 housed in the Palaeontology Section of the National Museums of Kenya, Nairobi ( Fig. 1a ) discovered during a field mission led by Meave Leakey in 1994. 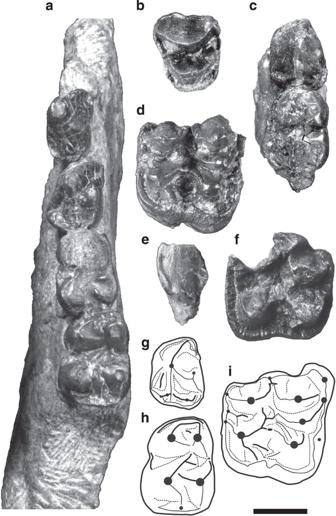Figure 1: Fossil remains ofEpirigenys lokonensisnov gen nov sp from late Early to early Late Oligocene of Lokone. (a) Left hemi mandible with P/3-M/2 (KNM-LH 30375, holotype) in dorsal view. (b) Left P4/ (KNM-LH 10298) in occlusal view. (c) Left P/4-M/1 (the fragmentary M/2 is not figured here; KNM-LH 11645) in occlusal view. (d) Right M3/ (KNM-LH 11650) in occlusal view. (e) Right I/1 (KNM-LH 51633) in lingual view. (f) Left M2/ (KNM-LH 58510) in occlusal view. (g) Drawing of the P/4 of KNM-LH 11645 in occlusal view. (h) Drawing of the M/2 of KNM-LH 30375 (holotype) in occlusal view. (i) Composite scheme of the upper molar occlusal morphology reconstructed from known parts of upper M2/ and M3/. Figure 1: Fossil remains of Epirigenys lokonensis nov gen nov sp from late Early to early Late Oligocene of Lokone. ( a ) Left hemi mandible with P/3-M/2 (KNM-LH 30375, holotype) in dorsal view. ( b ) Left P4/ (KNM-LH 10298) in occlusal view. ( c ) Left P/4-M/1 (the fragmentary M/2 is not figured here; KNM-LH 11645) in occlusal view. ( d ) Right M3/ (KNM-LH 11650) in occlusal view. ( e ) Right I/1 (KNM-LH 51633) in lingual view. ( f ) Left M2/ (KNM-LH 58510) in occlusal view. ( g ) Drawing of the P/4 of KNM-LH 11645 in occlusal view. ( h ) Drawing of the M/2 of KNM-LH 30375 (holotype) in occlusal view. ( i ) Composite scheme of the upper molar occlusal morphology reconstructed from known parts of upper M2/ and M3/. Full size image Hypodigm All the referred material is housed in the Palaeontology Section of the National Museums of Kenya, Nairobi. All the isolated material recovered from the three contemporaneous localities are biometrically and morphologically congruent with intraspecific variations in anthracotheres. The association of upper teeth and lower dental row is further motivated by size and occlusion match, as well as by a common dental pattern (massive and bulbous teeth with relatively short crests, thick enamel and relatively flat wear facets) not observed until now in other bothriodontines (see Supplementary Note 2 ). KNM-LH 10270 (Loc. 2): left dP4/; KNM-LH 10298 (Loc. 2, Fig. 1b ): left P4/; KNM-LH 11604 (Loc. 13): frag. left M/3; KNM-LH 11608 (Loc. 1): frag. left lower molar (trigonid); KNM-LH 11609 (Loc. 1): fragmentary upper molar; KNM-LH 11633 (Loc. 13): fragmentary of right M2-3/; KNM-LH 11642: left M1/ or M2/ (ref. 19 ); KNM-LH 11644 (Loc. 13): left dP4/; KNM-LH 11645 (Loc. 13, Fig. 1c ): left P/4-M/2; KNM-LH 11646 (Loc. 13): distal part of left M/3; KNM-LH 11647 (Loc. 13) frag left upper molar; KNM-LH 11650 (Loc. 13, Fig. 1d ): right M3/; KNM-LH 46214 (Loc. 1/2, 1995): probable left M2/; KNM-LH 47587 (Loc. 1/2, 1995): right fragmentary upper molar; KNM-LH 47845 (Loc. 1/2, 1994): distal part of left P/4; KNM-LH 47846 (Loc. 1/2, 1994): probable right M1/; KNM-LH 47847 (Loc. 1/2, 1994): frag. right M/2; KNM-LH 51633 (Loc. 1, Fig. 1e ): right I/1; KNM-LH 58510 (Loc. 13, Fig. 1f ): left M2/. Type locality and horizon Lokone Hill area near Loperot in the Lokichar basin, West Turkana District, Kenya. Loc. 1, 2 and 13 (GPS coordinates: 2°22′N and 35°57′E) situated in the Lokone Sandstone Formation are contemporaneous and have been dated from the late early Oligocene to the early late Oligocene [19] . Diagnosis Medium-sized bothriodontine. The following characters are unique within bothriodontines, differing notably from those of Bothriogenys , and shared with Hippopotamidae: developed cingular structures including high cingulid on labial side of P/3, presence of cingulid lingual to entostylid and high distal cingulid on P/4, high lingual cingulum on upper molars; strong and complex lower premolars with hypoconid on P/4, biconvex occlusal shape of premolars, developed post- and endoprotofossids, a short endoprotocristid; P4/ with mesial and distal accessory cusps; bunodont molars with rounded cusps, inflated crests (for example, prehypocristid in transverse valley of lower molars) and shallow valleys; presence of an entostylid on lower molars, and a groove separating preparacrista and parastyle. Enamel microstructure similar to that of Kenyapotamus , except for lacking inter-row sheet in inner part. Features shared with Bothriogenys but that are unknown in Hippopotamidae include the lack of an ectoprotofossid on P/4, the postmetacristid not orientated towards the centre of the tooth and the position of the distostylid on lower molars, mesio-distal ribs of labial cusps of upper molars less developed, the presence of two distal well-developed cristae on the protocone, the divided premetacristule, the lack of postmetafossule and the developed parastyle and mesostyle. Description E. lokonensis is a middle-sized anthracothere (see measurement in Supplementary Tables 1 and 2 ) with an estimated weight of 71–98 kg based on its M/1 area ( Supplementary Table 3 ; ref. 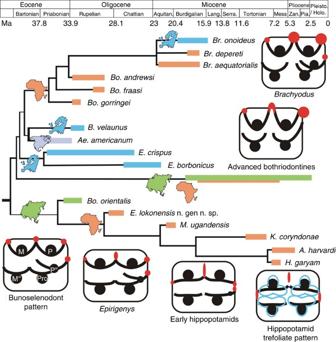Figure 3: Evolution of occlusal pattern in hippopotamoid. Part of the consensus tree (clade HB) replaced on the geologic time scale54and the geographic distribution, with the morphological evolution of the upper molar. Colour correspondence on upper molars: cristae and cusps in black, styles in red and wear pattern in blue. M, metacone; Mul, metaconule; P, paracone; Pro, protocone; Pul, paraconule. 25 ). Anterior teeth are only known by a spatulate I/1 ( Fig. 1e ). The structure of this incisor is similar to that of other bothriodontines (for example, Bothriogenys , Elomeryx and Bothriodon ) but it lacks the median lingual pillar. On the P4/, the preprotocrista and postprotocrista connect the mesial and distal cingulae, respectively, forming a mesio- and a distostyle ( Fig. 1b ). Both styles are developed in a way that mimics accessory cusps. This morphology differs markedly from that of Bothriogenys spp. where the postprotocrista never connects the distal cingulum and where no such styles development occurs. Upper molars are brachyodont with inflated cusps ( Fig. 1d,f and i ) and high cingula (approximately half the height of unworn cusps). Species of Bothriogenys display shallower cingula and the condition in E. lokonensis appears closer to that observed in Kenyapotamus coryndonae . Cristae are rather blunt and transverse valleys are not as deep as in Bothriogenys . The ribs of the labial cusps are inflated and not pinched due to the mesio-distal elongation of the cristae. It markedly differs from the crescentic cristae observed in Bothriogenys . In labial view unworn cusps are rounded. The postprotocrista is weakly developed compared with the postectoprotocrista that extends towards the transverse valley and reaches the premetacristule. There is a secondary postectoprotocrista mainly developed at the base of the protocone and in the transverse valley that is in the same lingual position as the postectoprotocristae of K. coryndonae [10] . The transverse valley is blocked at this level by the junction of these cristae. This junction is shallower in Bothriogenys spp. The mesial end of the premetacristule develops as a small conule. A short enamel fold occurs between the ecto- and the premetacristule on KNM-LH11650, which is not observed in other anthracotheres. The postmetacristule joins the cingulum and forms a distostyle as in Bo. orientalis and Bo. rugulosus but unlike Bo. gorringei and Bo. fraasi , in which this crest joins the base of the metacone. The distostyle in Epirigenys is distal to the labial wall of the metaconule, instead of the metacone. Several accessory cristules varying in size between teeth occur labially to the postmetacristule; they create additional minute wear facets and fill the longitudinal valley distally. The complexity of the crest network is markedly higher than in Bothriogenys , in which the valleys do not display such secondary structures. The preparacrista is slightly separated from the parastyle by a thin groove as in Kenyapotamus . The mesiostyle is very close to the parastyle. As in Bo. orientalis and Kenyapotamus , the labial cusps are not displaced lingually to the axis parastyle–metastyle contrary to more selenodont taxa ( Elomeryx , Microbunodon , African Bothriogenys and Brachyodus ). The mesostylar area is complex ( Fig. 1f,i ). The cingulum is developed and forms an ectostyle extended lingually into an ectocristyle. The postparacrista and premetacrista connect the lateral side of this cristyle that runs through the transverse valley. This pattern considerably differs from that seen in Elomeryx and other bothriodontines that lack the ectocristyle, and is similar to that observed in Bo. rugulosus and in Anthracotherium spp., suggesting a possible plesiomorphic condition. 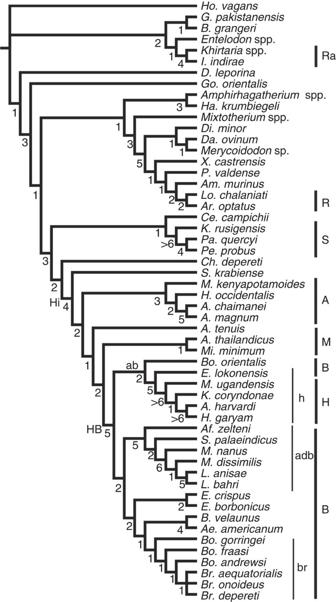Lower premolars are similar in size with those of Bo. Figure 2: Phylogenetic relationships of hippopotamoid. Consensus tree of the cladistic analysis obtained from the two most parsimonious trees (980 steps, CI=0.22, RI=0.61). A, Anthracotheriinae; ab,Bo. orientalis,E. lokonensisand Hippopotamidae; adb, advanced Bothriodontinae; B, Bothriodontinae; br,Brachyodusclade; H, Hippopotamidae; h,E. lokonensisand Hippopotamidae; HB, Hippopotamidae+Bothriodontinae; Hi, Hippopotamoidea; M, Microbunodontinae; R, Ruminantia; Ra, Raoellidae; S, Suoidea. Values below the branches are Bremer indices. gorringei ( Supplementary Table 2 ) but their lingual side is convex instead of concave ( Fig. 1a,c and g ). This feature is similar in lower premolars of kenyapotamines, microbunodontines, and anthracotheriines; it distinguishes them from those of known Bothriogenys and other bothriodontines. The lower premolars of Epirigenys are low and broad with cingulids that ascend the sides of the crown and form lateral V-shaped pillars. This structure, which is well-marked on the labial and lingual sides, forms edges comparable to accessory cristids. This is not observed on the labial side of lower premolars in Bothriogenys and is only slightly expressed on their lingual sides. Moreover, the presence of accessory cristids implies the development of post- and endoprotofossids, a pattern that has also been described in hippopotamids, including early kenyapotamines and Morotochoerus [10] , [11] . The preprotocristid is curved mesiolingually as in hippopotamids and other bothriodontines [10] . The endoprotocristid originates at the protoconid apex and joins the high lingual cingulid (half of the cuspid height) to form a large entostylid. The short endoprotocristid considerably differs from the long and curved endoprotocristid of Bothriogenys and Brachyodus . The P/4 is proportionally wider than in any species of Bothriogenys ( Supplementary Table 2 ). The lingual and distal cingulids are not connected whereas they are continuous in Bothriogenys and Brachyodus . This unusual morphology might be related to the height of the cingulid on both lateral sides of the cuspid and on the distal shelf. There is a small postectoprotocristid between the postprotofossid and the labial cingulid that is observed only in Morotochoerus ugandensis and one specimen of K. coryndonae . There is an incipient hypoconid close to the postprotocristid in the same position as in Kenyapotamus (for example, KNM-NA 194). The distal cingulid is broader and more developed than in Bothriogenys . The lower molars display low cuspids ( Fig. 1a,h ). The valleys are shallow, favoring an early connection between lingual and labial cuspids when worn. Therefore, little wear can lead to a lophid-like pattern, which is exceptional in anthracotheres but observed in kenyapotamines. The M/2s of Epirigenys are comparatively shorter and wider than those of Bothriogenys , and more similar in this regard to hippopotamids. The endometacristid is present and is lined by a deep premetafossid. This cristid is absent in Brachyodus and Bo. andrewsi . The posthypocristid is curved and joins the distostylid without any contact with the postentocristid. This pattern considerably differs from what is observed in other bothriodontines. The longitudinal valley of the talonid is poorly expressed and only a slight wear creates a large facet that includes the hypoconid and entoconid. An entostylid is present which is unknown in other anthracotheres (except Anthracotherium ) but frequent in hippopotamids [10] . A cingulid occurs at the labial end of the transverse valley and forms a minute ectostylid. The distal cingulid is high compared with the mesial one and is leveled with the distal longitudinal valley. A median distostylid is well-marked on the distal cingulid. The dental enamel Schmelzmuster of molar presents few inner radial enamel and is almost exclusively represented by Hunter Shreger Band zone. The Hunter Shreger Band are bent, thin and of regular aspect. The described enamel microstructure ( Supplementary Note 3 , Supplementary Fig. 2 ) is similar to that of early bothriodontines and Kenyapotamus [26] . Phylogenetic analysis The proposed phylogeny is highly homoplastic and well-structured (Consistency Index=0.22; Retention Index=0.61). We obtained two trees that differ in the resolution of the relationships between the three species of Brachyodus ( Supplementary Data 2 , Supplementary Fig. 16 ). In the strict consensus topology ( Fig. 2 ), the Hippopotamoidea ( sensu ref. 24 , that is, including anthracotheres and Hippopotamidae) are monophyletic. This node (Hi in Fig. 2 ) is supported by 10 non-ambiguous characters such as the presence of a preentocristid (51 1 ) and a complete ectohypocristulid on M/3 (67 2 ). Most of the characters that unambiguously define this clade correspond to dental structure features (crests and grooves) of molars. In this analysis, Siamotherium krabiense appears as the basalmost hippopotamoid. Anthracotheriinae forms a clade corresponding to the first offshoot (A in Fig. 2 ). This is congruent with previous known phylogenies of anthracotheres, for example, ref. 27 ; in addition our analysis places the Asian Myaingtherium kenyapotamoides into this sub-family. This position is in agreement with previous cladistic results [28] , but contradicts close relationships between M . kenyapotamoides and the Miocene African Kenyapotamus [28] . The clade HB (Bothriodontinae+Hippopotamidae; Fig. 2 ) is well-supported and congruent with previous phylogenetic hypotheses, for example, refs 29 , 30 . We noted 12 non-ambiguous traits including two non-homoplastic apomorphies: the presence of ectocristylids (65 1 ) and the bent orientation of Hunter–Schreger Bands (155 1 ). Most of the characters defining this clade correspond to enamel microstructure and premolar structures. Figure 2: Phylogenetic relationships of hippopotamoid. Consensus tree of the cladistic analysis obtained from the two most parsimonious trees (980 steps, CI=0.22, RI=0.61). A, Anthracotheriinae; ab, Bo. orientalis , E. lokonensis and Hippopotamidae; adb, advanced Bothriodontinae; B, Bothriodontinae; br, Brachyodus clade; H, Hippopotamidae; h, E. lokonensis and Hippopotamidae; HB, Hippopotamidae+Bothriodontinae; Hi, Hippopotamoidea; M, Microbunodontinae; R, Ruminantia; Ra, Raoellidae; S, Suoidea. Values below the branches are Bremer indices. Full size image Hippopotamidae form a clade (ab, Fig. 2 ) with Bo. orientalis and the new genus from Kenya. The sister group of clade ab is formed by the rest of the bothriodontines (B in Fig. 2 ), the latter grouping being moderately supported. Only advanced bothriodontines received a good support (node adb in Fig. 2 ), whereas the relationships between Elomeryx , Bothriodon and Bothriogenys remain fragile, in congruence with previous results, for example, ref. 27 . Yet, we obtained the successive branching of Bo. gorringei , Bo. fraasi, Bo. andrewsi and Brachyodus (node br in Fig. 2 ) as proposed by Black [31] . Consequently, the genus Bothriogenys is polyphyletic in our analysis. Eight non-ambiguous characters support the clade ab. Most of the characters defining this clade concern styl/id(es) pattern. The sister-group relationship between Epirigenys and Hippopotamidae (node h in Fig. 2 ) is well-supported by 10 non-ambiguous synapomorphies. One of them is non-homoplastic and based on premolar cingulid development (24 1 ). For at least three characters, Epirigenys presents features that might represent intermediate states between basal representatives of the HB clade (such as Bothriogenys ) and Hippopotamidae (26 0 , 43 1 , 44 1 ). Most of the characters defining this clade correspond to cingular structure and premolar morphology. The clade Hippopotamidae (node H on Fig. 2 , including Morotochoerus , Kenyapotamus and Hippopotaminae) is defined as a well-supported node, as in the study of Orliac et al. [11] We found 10 non-ambiguous synapomorphies and 11 ambiguous ones, the latter related to the scarcity of material attributed to the basalmost hippopotamid, M . ugandensis . Most of the characters defining this clade correspond to profound modifications of the molars towards a more bunodont pattern. These modifications have already been described by Orliac et al. [11] A maximum-likelihood tree obtained from the same matrix ( Supplementary Data 3 ) differs in: (1) the position of G. orientalis , (2) a clade gathering Bothriogenys , Brachyodus , the Hippopotamidae and E. lokonensis , and (3) the position of Elomeryx as stem advanced bothriodontines. This probabilist approach provides a result therefore more congruent with a previous phylogenetic hypothesis for Bothriodontinae [27] . In both case it also strongly supports the relationships between E. lokonensis and Hippopotamidae as well as the relationships of this clade with Bothriogenys . Despite advances in studying the record of early hippopotamids [10] , [11] , [32] , recent literature considering fossil data still inconsistently depicted their extrafamilial affinities, alternately favouring Suina, cebochoerids, ‘palaeochoerids’ or anthracotheres, for example, refs 1 , 2 , 4 , 5 , 7 , 8 , 10 , 11 , 26 , 33 . Some cladistic analyses considering an extended array of fossil taxa including basal hippopotamids and anthracotheres [4] , [10] , [11] , [24] , [29] , [30] supported a hippopotamid emergence within anthracotheres (‘anthracothere hypothesis’). However, these works proposed various anthracothere clades for alternative rooting of the Hippopotamidae: Anthracotheriinae, crown bothriodontines ( Merycopotamus and Libycosaurus ), advanced bothriodontines (including, for example, Sivameryx ) or archaic bothriodontines (for example, Bothriogenys ). These clades differ markedly in their degree of selenodonty, their ecologies and their spatiotemporal distributions, implying very different evolutionary and biogeographical scenarios for example, refs 2 , 34 . The discovery of Epirigenys greatly improves this condition, because it has been demonstrated to be a hippopotamoid displaying a functionally intermediate combination of characters, echoing the cetacean fossil discoveries celebrated by Gatesy [1] . Our phylogenetic study allows formal identification of the archaic bothriodontines as stem group of the Hippopotamidae (in accordance with some of the hypotheses discussed in refs 10 , 11 , 26 ). First, this placement unveils the complete evolutionary changes that led to the hippopotamid dental morphology. Second, it supports a single scenario explaining the biogeographical history of the hippopotamid emergence. Finally, it is an important step towards the resolution of relationships between basal cetancodonts. The evolution of the unique hippopotamid dental morphology has been historically viewed as a difficulty for each competing hypotheses on hippopotamid origins, for example, refs 35 , 36 . An emergence from bothriodontines (ref. 2 : Fig. 3 ) implied a moderately to markedly selenodont dental ancestry. In this context, Boisserie and Lihoreau [34] suggested that (1) this transition, requiring the mesio-distal reorientation and shortening of cristae, may have been relatively easy given the significant effects of some limited genotypic alterations on mammalian cusp morphologies, and (2) dental enamel thickening may also have played a role in shaping the hippopotamid dental pattern. The subsequent confirmation of Kenyapotamus and recognition of Morotochoerus as early hippopotamids [10] , [11] indicated that progressive paraconule reduction, reorientation of the cristae and migrations of the para- and metastyles took place in Miocene hippopotamids. Figure 3: Evolution of occlusal pattern in hippopotamoid. Part of the consensus tree (clade HB) replaced on the geologic time scale [54] and the geographic distribution, with the morphological evolution of the upper molar. Colour correspondence on upper molars: cristae and cusps in black, styles in red and wear pattern in blue. M, metacone; M ul , metaconule; P, paracone; Pro, protocone; P ul , paraconule. Full size image The identification of Epirigenys anchors the Hippopotamidae within a group of bothriodontines that displays a bunoselenodont dental pattern with relatively moderate stylar developments. Epirigenys has pentacuspidate upper molars, marked styles and distally closed trigonids, features that are typical of archaic bothriodontines such as Bothriogenys . In addition, the molar cusp/id pattern of Epirigenys is close to that of the earliest hippopotamids ( Morotochoerus ) in displaying thick cingula/ids, swollen cristae/ids, multiple secondary cristae/ids, shallow and obstructed valleys, moderately curved labial cristae, a parastyle disjoint from the preparacristae and relatively small styles/ids. In addition to this mosaic of molar features, Epirigenys displays low, massive and complex lower premolars as in early hippopotamids. This indicates that the dental evolution of Hippopotamidae from their bothriodontine ancestors was essentially achieved through combining: (1) the reorientation of crista/ids also observed in early hippopotamids; (2) stylar reduction; (3) a disconnection and an elongation of the postmeta- and postprotocristids distally opening the trigonid. These simple dental modifications contrast with the heavier dental changes required by alternative hypotheses, notably that of a hippopotamid emergence from advanced bothriodontines with derived selenodonty (for example, refs 29 , 35 , 37 , Fig. 3 ; 64 additional steps for the alternative hypothesis with Hippopotamids merging from advanced bothriodontines, sister group of Libycosaurus and Merycopotamus ). These results warrant a reassessment of two dental homologies and related nomenclature previously applied to the Hippopotamidae. First, Hippopotamidae display only one distal crista on the protocone directed towards the centre of the crown and often reaching the premetacristule. This crista is identified as the postprotocrista [10] . In Epirigenys and Bothriogenys , the postprotocrista is mesially flanked by a long postectoprotocrista in a similar position ( Fig. 3 ). The situation in Morotochoerus suggests that the crista found in Hippopotamidae could actually be the postectoprotocrista, the postprotocrista being reduced or even missing ( Fig. 3 ). In this case, Kenyapotamus might have occasionally developed a second, small and mesially oriented postectoprotocrista. This hypothesis should receive further support from the fossil record prior to full acceptance. Second, in bothriodontine lower premolars including those of Epirigenys , there is a strong elevation of the lingual cingulid that is an entostylid according to Boisserie et al. [10] In Epirigenys , the entostylid is stronger and more mesially positioned than in Bothriogenys , recalling in this the lingual cuspid observed in Hippopotamidae ( Fig. 3 ). However, in Kenyapotamus and especially in Hippopotaminae, this cuspid is often, although not always, mesially lined by a low cingulid, and is identified as a metaconid [10] . This was not observed on the limited specimen samples attributed to Epirigenys and Morotochoerus . Our observations and phylogenetic results strongly suggest that a secondary cingulid developed in later hippopotamids, the bothriodontine entostylid and the hippopotamid (secondary) metaconid being probably homologous. This hypothesis should be included in future phylogenetic analyses of the Hippopotamoidea. It should be noted that we used the previous nomenclature throughout this contribution. Previous studies led to propose at least two possible biogeographical scenarios for hippopotamid emergence [10] , [11] . However, the discovery of Epirigenys can help to favour only one scenario. Epirigenys , dated from the late early Oligocene or early late Oligocene [19] , is related to a group of archaic bothriodontines that expanded from Asia to Africa as early as the latest Eocene [21] ( Fig. 3 ). The oldest confident occurrence of Bothriogenys sp. in Africa is from the Fayum, Egypt (L25, Dir Abu Lifa Member of the Qasr el Sagha Formation [38] ). It can be noted that previous claims of a somewhat older occurrence at Bir el Ater, Algeria [39] was not confirmed by a re-examination of the material housed at the University of Oran. The dispersion phase of Bothriogenys may have been complex. Bothriogenys was relatively diverse in southeastern Asia during the late Eocene [40] , [41] , [42] . This diversity is echoed at the Fayum during the early Oligocene with two different genera of archaic bothriodontines [21] , [22] : Bothriogenys , represented by four species, and the monospecific genus Qatraniodon . In our opinion, a third archaic bothriodontine may be represented by an isolated tooth from the Fayum, initially attributed to ‘ Rhagatherium ’, see ref. 31 . The occurrence of Epirigenys at the early/late Oligocene transition in Lokone implies the presence in Africa of another lineage during the early Oligocene. Its affinities with Bo . orientalis from southeastern Asia rather than with Bothriogenys from the Fayum ( Fig. 3 ) suggest that the African diversification of the archaic bothriodontines occurred through multiple waves during the latest Eocene and the early Oligocene. Such a complex scenario would not be unique to anthracotheriids, several dispersal events from southeastern Asia to Africa having also been proposed for Eocene primates [43] , [44] and rodents [45] . According to our results, the subsequent evolution of African archaic anthracotheriids followed two main paths: (1) the branch that led from the Fayum species of Bothriogenys to the early Miocene Brachyodus ( Fig. 3 , in agreement with ref. 22 ); and (2) the branch of Epirigenys , eventually leading to the Hippopotamidae ( Fig. 3 ). Isotopic and morphological evidence suggests that the former lineage had semiaquatic habits throughout its evolutionary history [46] , [47] . These ecological conditions are also documented for fossil and extant hippopotamines [48] , and suggested by some isotopic results for Kenyapotamus [49] . In fact, the dispersal(s) of Asian archaic bothriodontines to insular Africa might have been favoured by semiaquatic adaptations, possibly a primitive condition for this group. However, both clades differ strongly in their dental evolution and in their outcome ( Fig. 3 ). Contrary to the progressive reduction of selonodont features in the hippopotamid clade, the selenodonty of the Fayum Bothriogenys was enhanced in Brachyodus that developed extremely enlarged styles ( Fig. 3 ). This latter genus included several large species and spread to Eurasia, but it became extinct before the middle Miocene, relatively soon after the dispersal of Asian advanced bothriodontines (for example, Sivameryx ) to Africa ( Fig. 3 ). Competition with those migrants, also displaying advanced selenodonty, might have been a significant factor in the extinction of the clade Bothriogenys – Brachyodus . During most of the Miocene, the hippopotamid lineage remained quite discrete, flourishing at the end of the epoch. During the Plio-Pleistocene, it gave rise to 30–40 species, most of them often large body-sized and it expanded several times to Eurasia [50] . Hippopotamids are still represented by two extant African species, testifying to the longest evolutionary sequence of terrestrial cetartiodactyls in Africa. It should be kept in mind that this scenario may somewhat evolve, notably because the nodes describing the relationships within ‘Anthracotheriidae’ are not as robust as the clade Epirigenys +Hippopotamidae and the clade of advanced bothriodontines. In particular, the paraphyly of Bothriogenys requires further confirmation and, if invalidated, it might lead to a simplification of the above presented scenario, notably regarding the initial phase of expansion from Asia to Africa. In addition, it should be noted that these interpretations are mostly based on dental evidence, and that the future integration of cranial and postcranial features in the context of broader-scale analyses, beyond the scope of this contribution, should be important in validating these hypotheses. Furthermore, the relationships within the outgroup should be further investigated in the future, notably with regard to the paraphyly of Cetruminantia obtained here—contra molecular phylogenies. This point should prove important in future works, first to focus on phylogenetic relationships potentially rooting archaic bothriodontines back to the early Eocene, and second to test if it might also affect relationships in the ingroup. The rooting of Hippopotamidae within archaic bothriodontines through a transitional form reduces previous morphological and biogeographical uncertainties on the anthracothere hypothesis. It also definitely strengthens the deep nesting of Hippopotamidae within ‘Anthracotheriidae,’ urgently calling for the integration of these data in future analyses, including ‘total evidence’ ones. A better understanding of the relationships between early cetancodonts will help producing robust reconstructions of the last common ancestor between whales and hippopotamuses. This would also provide a comprehensive phylogenetic framework to investigate the evolutionary pattern of the terrestrial/aquatic transition within Cetancodonta: it will be significant to understand whether the aquatic adaptations emerge in Cetancodonta as a synapomorphy, as multiple independent acquisitions or as multiple acquisitions triggered by shared underlying factors. It is also required to understand the role of semiaquatic adaptations in opening new evolutionary avenues to the cetancodonts, through expansions to landmasses overseas as well as to the seas themselves. Material origin Part of the material described here has been collected during two field missions in the Lokone area led by M. Leakey in 1994 and 1995. It corresponds to six specimens extracted from Loc. 1 or Loc. 2. Then two other field missions have been led in the same area (Loc. 1, Loc. 2 and Loc. 13) by the Lokone project in 2007 and 2009 and 13 specimens of E. lokonensis have been collected. Tooth description Dental descriptions follow the nomenclature established by Boisserie et al. [10] ( Supplementary Note 1 ). Specimen measurements are available in Supplementary Table 1 . Enamel microstucture investigations We followed the methodology, nomenclature and comparative materials described in Alloing-Séguier et al. [26] Two thin sections were performed: a horizontal one and a vertical one ( Supplementary Note 3 , Supplementary Fig. 2 ). Phylogenetic analyses We performed a cladistic analysis of 54 cetartiodactyl taxa including 30 hippopotamoids, 3 suoids, 2 ruminants and 19 basal cetartiodactyls as outgroup ( Supplementary Methods ). We described 164 unweighted and unordered craniodental characters for which almost 83 are original ones ( Supplementary Methods , Supplementary Figs 3–15 ), others being included or modified from published data matrix (refs 10 , 11 , 24 , 26 , 27 , 29 , 30 , 51 ). All characters are parsimony informative. We performed a heuristic search (10,000 replications) using Paup 4b10 (ref. 52 ) on the complete matrix ( Supplementary Data 1 ) and obtained two most parsimonious trees of 980 steps. We calculated Bremer support for each node up to seven supplementary steps ( Fig. 3 ). More than one-third of the consensus tree nodes (40%) are relatively robust (Bremer index≥3). The tree 2 and the apomorphic list are given in Supplementary Data 2 and Supplementary Fig. 16 . A maximum-likelihood analysis was performed with RaxML v. 8.0.2 (ref. 53 ) on the same data matrix, but as RaxML does not accept polymorphism for morphological data, these were changed to the most common state in the systematic group ( Supplementary Data 3 ). Homacodon vagans was set as the outgroup. We performed 1,000 bootstraps to assess node supports ( Supplementary Fig. 17 ). The command used was: raxmlHPC-SSE3 -s EpirigenysML.txt -n EpirigenysML.out -f a -m MULTIGAMMA -K MK -#1000 -p $RANDOM -x $RANDOM. (Shell command to generate a random number). Nomenclatural Acts This published work and the nomenclatural acts it contains have been registered in ZooBank, the proposed online registration system for the International Code of Zoological Nomenclature (ICZN). The ZooBank LSID (Life Science Identifiers) can be resolved and the associated information can be viewed through any standard web browser by appending the LSID to the prefix ‘ http://zoobank.org/ ’. The LSID for this publication is: 0269941B-201A-4677-B65A-3F413387B3F4. How to cite this article: Lihoreau, F. et al. Hippos stem from the longest sequence of terrestrial cetartiodactyl evolution in Africa. Nat. Commun. 6:6264 doi: 10.1038/ncomms7264 (2015).